Studying electrons on curved surfaces by trapping and manipulating multielectron bubbles in liquid helium Investigations of two-dimensional electron systems (2DES) have been achieved with two model experimental systems, covering two distinct, non-overlapping regimes of the 2DES phase diagram, namely the quantum liquid phase in semiconducting heterostructures and the classical phases observed in electrons confined above the surface of liquid helium. Multielectron bubbles in liquid helium offer an exciting possibility to bridge this gap in the phase diagram, as well as to study the properties of electrons on curved flexible surfaces. However, this approach has been limited because all experimental studies have so far been transient in nature. Here we demonstrate that it is possible to trap and manipulate multielectron bubbles in a conventional Paul trap for several hundreds of milliseconds, enabling reliable measurements of their physical properties and thereby gaining valuable insight to various aspects of curved 2DES that were previously unexplored. Electrons near the surface of liquid helium experience an attractive force due to the finite polarizability of the bulk liquid, but they are prevented from entering into the bulk due to a potential barrier [1] of ~1 eV in magnitude; this results in the formation of a layer of electrons floating above the liquid surface. The different phases of this [2] and other [3] two-dimensional electron systems (2DES) is determined by the ratio (Γ) of the electrostatic potential to the electronic kinetic energy, where n is the areal charge density for the 2D layer embedded on a medium of dielectric constant ε r . Depending on the value of Γ 137, the system can behave as a Wigner solid [4] or as a fluid. However, for electrons above helium, the kinetic energy of the 2DES is always dominated by classical (thermal) fluctuations, as the thermal energy k B T is typically much larger than the maximum quantum kinetic energy . This limitation in E F is related to the maximum density (>2 × 10 13 m −2 ) achievable with electrons above bulk liquid helium ( 4 He), beyond which an electrohydrodynamic instability [5] of the charged interface is developed, resulting in the break-up [6] of the liquid surface into small (micron scale) charged cavities, known as multielectron bubbles (MEBs). Note the density of electrons above the surface of thin helium films can be significantly higher than what is achievable above bulk liquid helium. We discuss in detail the comparison between the 2DES on thin films and the MEBs in a later section. The electrons inside the MEBs repel each other to form a 2D layer close to the inside surface of the bubble, forming a unique 2DES on a curved surface. The equilibrium radius ( R 0 ) of the bubble for a spherical MEB containing Z electrons is obtained by minimizing the total energy, given by where σ is the surface tension of liquid helium and P is the excess pressure of the outside with respect to the inside of the bubble. This yields an equilibrium radius of at P =0 resulting in a surface density given by For Z =10 2 –10 9 , n can vary between 3 × 10 15 and 1.5 × 10 13 m −2 , such that the maximum kinetic energy of the 2DES is dominated by quantum fluctuations, given by E F ~9 k B . In case of any applied pressure ( P >0), the surface densities can be made even higher, corresponding to a scenario overwhelmingly dominated by quantum fluctuations, similar to silicon metal-oxide-semiconductor devices or GaAs heterostructures, where the 2DES is always in a quantum liquid phase. The large tunability of surface density in MEBs can therefore provide a unique 2DES, whose thermodynamic phases, in principle, can range all the way from classical fluid-Wigner solid phases to much beyond the quantum solid–liquid melting transition. An equally interesting feature of the MEBs is that the electrons reside on the curved and flexible wall of the bubble, pushed against the surface by very large electric fields generated by the other electrons. Taken together, this unique system is expected to show various interesting physical phenomena, including quantum melting [7] , [8] and sonoluminescence [9] , but has been subject to limited experimental investigation [6] , [10] , [11] , [12] , [13] , [14] , [15] . This is probably because the previous studies mostly comprises the generation and subsequent annihilation of the MEBs in a charge collection electrode, thereby providing limited scope for measurement of their physical properties. As we demonstrate in this paper, it is possible to trap MEBs in a conventional ion trap in liquid helium, so as to manipulate and measure their physical properties over a duration that is significantly longer than what has been achieved before. In particular, we have estimated their size and charge in a non-destructive measurement, which also allowed us to determine their natural lifetimes, thereby paving the way towards more detailed investigations of this rich 2DES. Experimental setup In the experiments described here, we have used confined field emission above the liquid surface to generate [15] MEBs. A voltage pulse of few kV and duration 30–50 ms was applied to a sharp tungsten tip placed inside a plastic tube above the helium surface. At temperatures below the λ -point ( T λ =2.17 K), the liquid surface became unstable due to the application of the voltage pulse, resulting in the formation of large bubbles (size approximately a few hundred micrometres). These bubbles shrank to a size below a few micrometres in a time scale of a few milliseconds and could not be detected visually thereafter. Qualitatively similar phenomenon was observed above T λ , where a large number of bubbles of sizes ranging in diameter from ~10 to 100 μm were formed due to the instability of the liquid surface, and which could be observed for significantly longer times. Most of the experiments reported in this article were carried out at around 2.5 K, that is, above T λ . Following their generation, the bubbles drifted downward due to the presence of the negative voltage on the field emission tip and entered the 2D Paul trap (see Methods for more details on the injection process), shown schematically in Fig. 1a . Typically, we applied sinusoidal voltages of few kV at frequencies of few hundred Hz to the rods, and around −1 k V dc to the end rings for confining the MEBs in the axial direction. It is important to note that operating parameters (voltage and frequency) of our trap were significantly different from the typical parameters used in the ion trap experiments, which is essentially due to the finite drag on the MEBs due to the viscosity of liquid helium as opposed to the frictionless motion of trapped ions in vacuum. The standard method of estimating trap parameters is based on frictionless conditions, which results in the equations of motion being reduced to the well-known Mathieu equations, cannot be used in the present scenario, thereby necessitating a numerical simulation for estimating the correct trap parameters. The results of the numerical calculations for estimating the electrical fields in the trap region are shown in Supplementary Fig. 1 , while the details of the numerical simulations to predict the motion of MEBs under various trap conditions are given in Supplementary Note 1 . Another important difference of this system from common ion traps stems from the large effective mass of the MEBs, which is proportional to the mass of the displaced fluid. For an MEB of radius 10 μm, this corresponds to a mass of ~10 14 times the mass of a helium atom. Accordingly, the MEBs could not be trapped with operating conditions used in typical ion traps, as shown in Supplementary Fig. 3 . 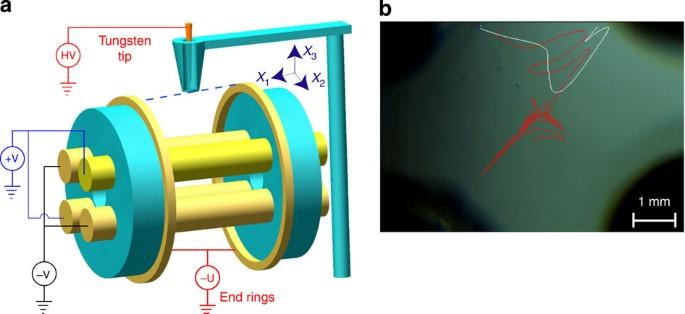Figure 1: Trapping of MEBs and their typical trajectories. (a) Schematic of the experimental setup to generate and trap MEBs. Field emission from the tungsten tip charges the liquid surface; the four horizontal metal rods of diameter 3 mm and separated diagonally by 5 mm provide the trapping electric field while the end rings confine the MEBs to the trap centre. Dotted line indicates the level of liquid helium. (b) Trajectory for a stably trapped MEB (red), along with that of an MEB, which rose up due to buoyancy and left the trap (white).The view of the camera was along theX1axis, that is, along the length of the rods. Figure 1: Trapping of MEBs and their typical trajectories. ( a ) Schematic of the experimental setup to generate and trap MEBs. Field emission from the tungsten tip charges the liquid surface; the four horizontal metal rods of diameter 3 mm and separated diagonally by 5 mm provide the trapping electric field while the end rings confine the MEBs to the trap centre. Dotted line indicates the level of liquid helium. ( b ) Trajectory for a stably trapped MEB (red), along with that of an MEB, which rose up due to buoyancy and left the trap (white).The view of the camera was along the X 1 axis, that is, along the length of the rods. Full size image We could image three types of objects in this experiment with a fast camera running at ~20,000 frames per second: uncharged bubbles, which did not respond to the oscillating electric fields, and which rose up due to buoyancy and left the trap; unstably trapped MEBs, which responded to electric fields, but typically left the trap within few to tens of milliseconds; stably trapped MEBs, which could be observed for a much longer duration (approximately hundreds of milliseconds). Many of the stably trapped MEBs could not be observed after some time, simply because the depth of focus of the optical system was less than the size of the trap region. However, certain MEBs stayed in the trap, shrank in size and then disappeared; this will be discussed in greater detail later. The trajectory of a stably trapped MEB and an MEB that could not be trapped has been shown in Fig. 1b . See also the corresponding Supplementary Movie 1 . It is noteworthy that during the course of our experiments, we have observed various other types (shapes) of trajectories (see Supplementary Fig. 4 ) as well. Analysing trajectories of MEBs The successful trapping of the MEBs allowed us to measure their charge and radii independently in a non-destructive manner. Note that we could not use standard light-scattering techniques to estimate the size of the MEBs, due to the interference from the light scattered by the constant bubbling liquid above T λ . Our method was based on imaging and analysing their trajectories under various forces, as shown schematically in Fig. 2b . Initially, the MEBs were trapped by applying sinusoidal voltages to the rods, which allowed us to differentiate between the oscillating MEBs and the uncharged vapour bubbles. Subsequently, we turned off the trap for a short duration such that the MEBs drifted upward, which allowed us to estimate their radii by analysing the trajectories under the action of buoyancy alone. Unless the MEBs were very close to the rods, the effect of the electric field due to image charge could be neglected. In our analysis, the MEBs were assumed to be spherical with radius R 0 and charge Q=Ze , having a hydrodynamic mass . Typical example of a best fit of R 0 (14 μm) obtained by analysing the trajectory of a rising MEB is shown in Fig. 2a . The next step was to assume the same value of R 0 and to analyse the trajectory of the MEBs to estimate their charge Ze , during the time when the trap was on. The assumption of constant R 0 was reasonable, provided the trajectory was imaged immediately before or after the time of the buoyancy measurement. This assumption could be additionally verified by looking at the MEB images as well. The governing equation was given by: , where the terms in the right correspond to forces arising from the applied electric field ( E ap ), due to the electric field ( E im ) from the image charges induced in the rods, due to gravity (proportional to R 0 3 ) and due to the viscous drag, given by , where the drag coefficient C D can be obtained from literature [16] , [17] . The applied and the image charge-induced electric fields as a function of position within the trap were obtained from numerical calculations using analytical formula [18] , [19] and finite element calculations. It was not possible to fit longer trajectories with this simple model, as the continuously boiling liquid had a randomizing effect on the motion of the MEBs. As shown in Fig. 2 , the quality of the fit for charge was reasonable up to two cycles of the trajectory, with the best fit obtained for Z =2,160. In this regard, let us mention the confidence level with which the best fits for radius and charge were obtained. Based on the variation of least square error as a function of the fitting parameter, we estimate the radius measurement to be accurate within 10%. On the other hand, the fit for charge was highly sensitive to the assumed value of the radius and the quality of the fit had some variation at different times of the MEB trajectory. For the example shown in Fig. 2 , the best fit of the charge varied between 1,500 and 4,000 electrons ( Z =2,750±1,250); in general, the charge estimation was correct within an order of magnitude. 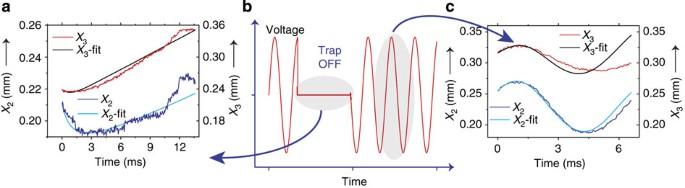Figure 2: Estimating charge and radius of a stably trapped MEB. (b) Results used to make a non-destructive measurement of the radius and the charge. Sinusoidal voltages of frequency 150 Hz and amplitude 3,000 V were applied to the rods, except for a brief period when the trap was turned off, thereby allowing the MEBs to rise up due to buoyancy. (a)X2–X3trajectories (red and blue) of the MEB due to buoyancy alone, along with the calculated trajectory (black and cyan) corresponding to the best fit of the radius (R0=14 μm). (c)X2–X3trajectories (red and blue) when the trap is on, along with the best fit of the charge (black and cyan), using the estimated value of radius (R0). Figure 2: Estimating charge and radius of a stably trapped MEB. ( b ) Results used to make a non-destructive measurement of the radius and the charge. Sinusoidal voltages of frequency 150 Hz and amplitude 3,000 V were applied to the rods, except for a brief period when the trap was turned off, thereby allowing the MEBs to rise up due to buoyancy. ( a ) X 2 – X 3 trajectories (red and blue) of the MEB due to buoyancy alone, along with the calculated trajectory (black and cyan) corresponding to the best fit of the radius ( R 0 =14 μm). ( c ) X 2 – X 3 trajectories (red and blue) when the trap is on, along with the best fit of the charge (black and cyan), using the estimated value of radius ( R 0 ). Full size image Measured radius and charge of trapped MEBs Based on the relation , the expected radius of an MEB containing 2,750 electrons was 0.5 μm, a value significantly smaller than the observed radius of 14 μm. We propose that the discrepancy was due to the presence of excess vapour inside the MEB, that is, vapour with a higher density than saturated vapour at the temperature of the liquid. Thus, the surface of the MEB was stabilized by three forces: outward pressure due to the excess vapour (Δ P ν ) and the layer of electrons pinned to the inside surface of the MEB, and the inward pressure due to the surface tension. Assuming the forces to be balanced, it was possible to estimate the amount of excess vapour inside the MEB, given by . For the example shown in Fig. 2 , this yields a value of Δ P ν ≈−35 Pa, which implies the vapour to be ~2 mK higher than the surrounding liquid at 2.7 K. The measured charge and radius for various MEBs are shown in Fig. 3 . It is interesting to note that the measured electron densities of the MEBs were close, but always less than the maximum density (~2 × 10 13 m −2 ) achievable above the surface of bulk liquid. This is probably related to the manner in which the MEBs were produced. On application of the voltage pulse, the field emission tip heated the liquid surface inside the plastic tube locally, thereby resulting in the formation of uncharged bubbles, which entered the trap due to the momentum generated at the onset of the surface instability. The MEBs were formed in the same manner; with the important difference that with MEBs, the charge residing on the liquid surface remained trapped inside the bubble beyond the onset of the surface instability, thus retaining almost the same surface charge density of the bulk interface. 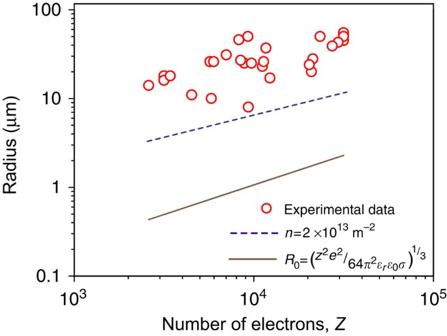Figure 3: Measured radius and charge of trapped MEBs. Results for the measured radii versus charge for different MEBs, following the procedure shown inFig. 2. The solid line corresponds to the theoretical radius versus charge for zero applied pressure. The dotted line corresponds to a surface electron density of 2 × 1013m−2, the density at which the surface of bulk liquid helium becomes unstable. Figure 3: Measured radius and charge of trapped MEBs. Results for the measured radii versus charge for different MEBs, following the procedure shown in Fig. 2 . The solid line corresponds to the theoretical radius versus charge for zero applied pressure. The dotted line corresponds to a surface electron density of 2 × 10 13 m −2 , the density at which the surface of bulk liquid helium becomes unstable. Full size image Increasing surface charge density of an MEB Trapping allowed the observation of MEBs over a significantly long duration, till they shrunk in size and could not be imaged any more (see Supplementary Movie 2 ). The shadow cast by an MEB on the imaging sensor to a good approximation was proportional to its extinction cross-section. The ratio of the extinction to the geometrical cross-section can be estimated from standard Mie theory calculations, while the radius of the MEB measured during the buoyancy measurements provided an accurate calibration. Together, this allowed us to estimate the variation of the radius of the MEB with time, that is, R ( t ). As shown in Fig. 4 , the rate of decrease of R ( t ) was highly nonlinear, with slow initial decrease leading to a sudden final collapse. 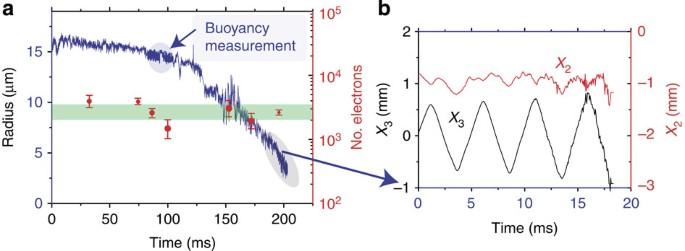Figure 4: Measurement of the radius of an MEB from generation to collapse. (a) Plot of the radiusR(t) as a function of time for a vanishing MEB, estimated from the shadow cast in the camera by the bubble. The values were scaled against the buoyancy-based measurement of the radius, as described in the text before. Also shown in red are the estimates of the number of electrons obtained by fitting the trajectory at certain time intervals (the value of error bars corresponds to the variation in the estimated number of electrons when the least square error of the fitting becomes 10% of the minimum), along with the bounds of the estimated number of electrons depicted by the green shaded region. (b)X2–X3trajectory of the MEB during the last three to four cycles before vanishing. Note the increase in amplitude of theX3trajectory as the size of the bubble reduced. We could not detect the MEB when the radius was smaller than 3 μm, a limitation posed by the contrast of the images obtained in our optical setup. Figure 4: Measurement of the radius of an MEB from generation to collapse. ( a ) Plot of the radius R ( t ) as a function of time for a vanishing MEB, estimated from the shadow cast in the camera by the bubble. The values were scaled against the buoyancy-based measurement of the radius, as described in the text before. Also shown in red are the estimates of the number of electrons obtained by fitting the trajectory at certain time intervals (the value of error bars corresponds to the variation in the estimated number of electrons when the least square error of the fitting becomes 10% of the minimum), along with the bounds of the estimated number of electrons depicted by the green shaded region. ( b ) X 2 – X 3 trajectory of the MEB during the last three to four cycles before vanishing. Note the increase in amplitude of the X 3 trajectory as the size of the bubble reduced. We could not detect the MEB when the radius was smaller than 3 μm, a limitation posed by the contrast of the images obtained in our optical setup. Full size image There could be multiple factors that stabilized the MEBs over hundreds of milliseconds. As predicted in several theoretical calculations [20] , [21] , [22] , [23] , [24] , [25] , [26] , the surface fluctuations of the MEBs, both radial and angular modes, are expected to play an important role; however, the finite viscosity of liquid helium above T λ could dampen the surface fluctuations significantly. Most importantly, the presence of the heated vapour inside the MEB is equivalent to applying a negative pressure at the outside of the bubble with respect to the inside ( P =Δ P ν <0), which could stabilize the MEB against surface oscillations. The low thermal conductivity of the liquid above T λ was responsible for the slow rate at which the heated vapour condensed, which could explain the slow initial decrease of the radius. An interesting question that raises itself is whether the charge of the MEB remained constant during its life cycle, as this can provide important insight into the mechanisms leading to the stability or instability of the MEBs against breaking into smaller MEBs, as well as predict the phase of the (curved) 2DES. During the course of our experiments at temperatures around 2.5 K, we have indeed observed certain MEBs, which break spontaneously into two or three smaller fragments, although the occurrence of these events were quite rare (~1%). For the result shown in Fig. 4 , we could not detect any smaller bubble being generated during its entire lifetime. To obtain a more quantitative estimate, we measured the charge at different instances by fitting the trajectory of the MEB over one cycle of the electric field modulation (150–200 Hz). We estimated the radius by analysing the images and assumed the radius to be constant during one cycle (~5–6 ms). This was a reasonable approximation, as the rate of change of radius was measured to be within 20 and 200 μm s −1 . As shown in Fig. 4 , the charge was found to remain constant (with bounds of the estimate between 2,000 and 3,500 electrons) during the entire time of our observations, as the MEB reduced from 16 to 3 μm. This was further supported by the observation that during the final 10 ms of its lifetime, the shrinking MEB showed a large increase in velocity. The oscillatory motion of the vanishing MEB was around the same position in the X 2 – X 3 plane (see Fig. 4b ), implying the effective electric forces were of similar strength, which meant the increase in amplitude was solely due to the reduced drag of the vanishing bubble. This large reduction of the radius of the MEB (with Z =2,750) from 14 μm to its equilibrium radius at zero pressure ( R 0 =0.5 μm), implies a maximum density of 8 × 10 14 m −2 , a value significantly higher than what can be achieved with electrons on the surface of bulk liquid helium. A system of great relevance to MEBs is that of charged helium films [27] , where electron densities >10 15 m −2 have been achieved [28] , [29] , [30] . The maximum achievable density in helium films is related to the minimum possible thickness of the film, which by itself is limited by quantum tunnelling of the electrons through the liquid film into the underlying substrate. On the other hand, the surface densities of MEBs can be significantly higher for bubbles with small , or made very large by application of pressure. As an example, consider an externally applied pressure of P =1 bar applied on an MEB with Z =2,750, which results in an equilibrium radius of 0.16 μm and a corresponding charge density ~8.7 × 10 15 m −2 . Pressure oscillations of similar [31] , [32] and much higher [33] magnitudes have been achieved in liquid helium with sound waves in recent years. Although both MEBs and helium films can be highly charged, a much bigger difference arises due to the intrinsic curvature of MEBs, which results in an extremely large pressing field on the electrons, pushing them deep into the inner surface of the bubble. Theoretical calculations on MEBs including such effects of curvature predict a unique phase described as a Wigner lattice of ripplopolarons, and the existence of an electron liquid phase as well. Interestingly, the theoretical calculations of the curved 2DES at zero pressure have predicted [7] the existence of the quantum liquid state at surface densities as low as 7.7 × 10 12 m −2 , a result that is significantly different from the corresponding value [28] reported for flat 2DES. We believe the investigation of such and various other novel aspects of curved 2DES may now be possible with trapped MEBs. In conclusion, trapping MEBs can open up new avenues in the study of 2DES, where the effects of curvature have been predicted to give rise to various novel phenomena [8] , [9] , [34] , [35] , [36] . The 2DES inside a single MEB can go through large changes in surface density under electric fields that are unattainable in any other system, and thereby provide access into aspects of 2DES phase diagram that has never been explored before. Furthermore, studying stability criteria of the MEBs can provide insight into the dynamics of charged droplets and bubbles, and mechanisms that affect their stability. It will be particularly interesting to determine the fate of an MEB beyond its collapse. Apart from a large number of single electron bubbles, there is a recent prediction [37] about the formation of stable bubbles containing four, six and eight electrons; we will investigate their possible existence in near future. Injection of MEBs into the trap The MEBs were created by applying a large negative pulse to the field emission tip during a time when zero voltages were applied to the trap rods. Owing to the negative potential on the tip and the negative charge of the MEBs, the bubbles were pushed downward away from the tip (against the force of buoyancy) and entered the trap region. At this instant, the tip was turned off and the voltage to the rods was turned on, thereby getting the MEBs trapped. To explain the process of injection in detail, we used a different experimental setup shown schematically in Fig. 5a , where the trap rods have been replaced with a copper wire, working as anode. For the experiment reported here, the anode was kept at zero voltage. We applied a negative voltage (~ few kV) of duration ~30 ms to the field emission tungsten tip, which results in the formation of a 2DES on the helium surface with subsequent breakage of the surface into MEBs. The bubbles move downward primarily because of the inertia of the unstable surface and subsequently due to the repulsion of the negatively charged MEBs by the tip kept at negative potential. As the voltage to the tip was increased to zero, the MEBs moved upwards due to buoyancy. This process is shown schematically in Fig. 5a and an experimentally obtained trajectory is shown in Fig. 5c (see also corresponding Supplementary Movie 3 ). 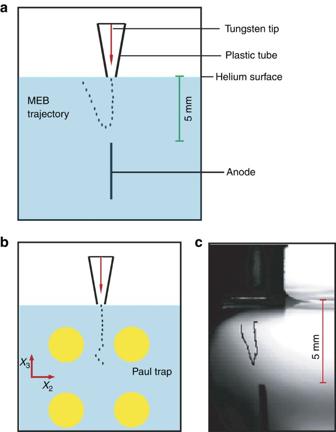Figure 5: Injection of MEBs into the trap. (a) Schematic of the experimental setup with an MEB drifting downward till the tip was at a negative potential, and its subsequent motion upwards due to buoyancy when the voltage to the tip was turned off. (b) Schematic of the process of injection of MEBs into the trap. The voltages to the rods were turned on and the tip was turned off, at the instant when the MEBs were inside the trap. (c) Experimentally obtained trajectory of an MEB following the idea discussed inFig. 1a. The images were taken fromSupplementary Movie 3. Figure 5: Injection of MEBs into the trap. ( a ) Schematic of the experimental setup with an MEB drifting downward till the tip was at a negative potential, and its subsequent motion upwards due to buoyancy when the voltage to the tip was turned off. ( b ) Schematic of the process of injection of MEBs into the trap. The voltages to the rods were turned on and the tip was turned off, at the instant when the MEBs were inside the trap. ( c ) Experimentally obtained trajectory of an MEB following the idea discussed in Fig. 1a . The images were taken from Supplementary Movie 3 . Full size image In the trapping experiments, the voltages to the rods were turned on at the instant the MEBs were in the trap region, while making the voltages applied to the tungsten tip increase to zero as well. This ensured successful injection and trapping of the MEBs, as shown schematically in Fig. 5b . How to cite this article: Vadakkumbatt, V. et al. Studying electrons on curved surfaces by trapping and manipulating multielectron bubbles in liquid helium. Nat. Commun. 5:4571 doi: 10.1038/ncomms5571 (2014).